Direct experimental observation of stacking fault scattering in highly oriented pyrolytic graphite meso-structures Stacking fault defects are thought to be the root cause for many of the anomalous transport phenomena seen in high-quality graphite samples. In stark contrast to their importance, direct observation of stacking faults by diffractive techniques has remained elusive due to fundamental experimental difficulties. Here we show that the stacking fault density and resistance can be measured by analyzing the non-Gaussian scatter observed in the c-axis resistivity of mesoscopic graphite structures. We also show that the deviation from Ohmic conduction seen at high electrical field strength can be fit to a thermally activated transport model, which accurately reproduces the stacking fault density inferred from the statistical analysis. From our measurements, we conclude that the c-axis resistivity is entirely determined by the stacking fault resistance, which is orders of magnitude larger than the inter-layer resistance expected from a Drude model. Graphite is known to be a semi-metal with a highly anisotropic electrical resistivity arising from the difference in effective mass of the conduction electrons moving along in-plane (ab-axis) and out-of-plane (c-axis) directions. While the experimentally measured in-plane resistivity and its temperature dependence behave as expected for phonon scattering being the dominant scattering mechanism, the out-of-plane resistivity ρ c is anomalously high even in high-quality samples and it exhibits markedly different scaling with temperature as compared to ρ ab (refs 1 , 2 , 3 , 4 , 5 , 6 , 7 ). The origin of the anomalous behaviour has remained a long-standing debated subject. It has been proposed that the anomalously high resistivity is caused by two-dimensional planar stacking fault defects acting as highly resistive barriers in the one-dimensional conduction path along the c-axis [8] , [9] , [10] . Such defects are expected to be randomly distributed along the c-axis with a theoretically predicted mean density in the order of 0.1 defects per nm [10] . Because of the high resistivity associated with stacking fault defects they have also been suggested as a decoupling mechanism for coherent electronic states, which are responsible for anomalous quantum transport behaviour observed in highly oriented pyrolytic graphite (HOPG) [11] , [12] , [13] . Despite the significance of the subject, the concept has remained speculative and lacks direct experimental verification. For example, an experimental measurement of important parameters such as the stacking fault density or the stacking fault resistance is missing. Here we report on an experimental study to directly address these points. A hallmark feature of stacking fault defects is the presence of high electrical resistance barriers associated with the randomly distributed defects. As a result, one expects to see characteristic non-Gaussian scatter of the c-axis electrical resistance, which is readily observable in structures containing only a small number of defects. Based on this concept, the electrical resistance of mesoscopic cylindrical HOPG pillars with the pillar axis pointing along the c-axis is measured, see Fig. 1a . There is a high probability that stacking fault defects extend across the entire pillar cross-section provided that the pillar radius r is less than the grain size of the sample, that is, r <1 μm. Hence, the randomly distributed defects act as a chain of series resistors, dominating the overall electrical transport along the pillar axis. Accordingly, the scatter of the measured pillar resistances is substantially non-Gaussian if the pillar height h is less than ~10 times the defects spacing, that is, h <100 nm. Here we show that this statistical fingerprint is indeed experimentally observed. From the measured statistics ,we infer a mean stacking fault distance in the order of 4 nm. We also measure non-linear current-versus-voltage (I/V) characteristics if the field strength exceeds 5 mV nm −1 . The non-linear characteristics can be perfectly fit to a thermally activated transport model with a mean spacing between the barriers of 3.9 nm consistent with the statistical analysis. The results are further corroborated by a model simulation, which accurately reproduces the non-linear conduction as well as the observed statistical scatter in the data. 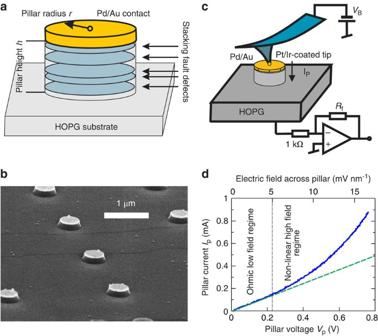Figure 1: Experimental procedures. (a) Schematic of a HOPG pillar with the pillar axis pointing along the crystallographic c-axis with randomly distributed stacking fault defects hallmarked by high resistance barriers for the current conduction along the c-axis. (b) Scanning electron microscopic image of 90-nm tall pillars fabricated on a HOPG substrate using an oxygen-reactive ion plasma etch and Pd/Au metal masks with a radius of 200 nm. (c) Schematic of the experimental set-up. (d) Typical current-versus-voltage characteristics measured on a 44-nm tall pillar with a radius of 300 nm. The measured current starts to deviate from the resistive dashed line as a threshold field of ~5 mV nm−1is exceeded. Figure 1: Experimental procedures. ( a ) Schematic of a HOPG pillar with the pillar axis pointing along the crystallographic c-axis with randomly distributed stacking fault defects hallmarked by high resistance barriers for the current conduction along the c-axis. ( b ) Scanning electron microscopic image of 90-nm tall pillars fabricated on a HOPG substrate using an oxygen-reactive ion plasma etch and Pd/Au metal masks with a radius of 200 nm. ( c ) Schematic of the experimental set-up. ( d ) Typical current-versus-voltage characteristics measured on a 44-nm tall pillar with a radius of 300 nm. The measured current starts to deviate from the resistive dashed line as a threshold field of ~5 mV nm −1 is exceeded. Full size image Experimental procedure The HOPG pillars with radii in the range 100–500 nm and with height in the range 22–90 nm were fabricated by means of dry plasma etching using Pd/Au metal mesas as self-aligned etch masks, see Fig. 1b and Methods section. The metal mesas also serve as electrical contacts to the top pillar surface, whereas the bottom contact is formed by the HOPG substrate. An atomic force microscope (AFM) was used to individually address the pillars by cold welding the Pt/Ir-coated tip to the Au surface of the metal mesas, see Fig. 1c . The electrical transport was characterized by measuring I/V characteristics. It was found that the I/V characteristics significantly deviate from a linear Ohmic behaviour if the field strength was larger than ~5 mV nm −1 , see Fig. 1d . This threshold field is typically not exceeded in macroscopic studies, which explains the lack of corresponding reports in the literature with the exception of refs 14 , 15 , reporting on mesoscale transport measurements in HOPG. Resistivity measurements We first examine the low field behaviour in the linear Ohmic regime. As anticipated by the stacking fault picture a huge scatter of the pillar resistance data is observed. To cope with the scatter, a median analysis (see Methods section) was applied for the data analysis. According to Ohm’s law the pillar resistance is given by which predicts that the resistance per unit height R P / h should scale inversely with the pillar area π r 2 , and the specific pillar resistance R P × π r 2 should scale linearly with the pillar height. This is indeed the case for the median average of the data as shown in Fig. 2a,b , respectively (note that the apparent deviation from the area scaling for 100-nm radius pillars in Fig. 2a is not statistically significant as explained in the Methods section). Therefore, we may use equation (1) to compute the c-axis resistivity from the pillar resistance data and we obtain a median value of ρ c =3.8 × 10 −3 Ω m. The non-Gaussian nature of the statistics governing the data scatter is clearly seen in Fig. 2b . The total scatter spans almost 2 orders of magnitude for the 22-nm tall pillars and a bit less than 1 order of magnitude for the 90-nm tall pillars. A robust measure for the data scatter is provided by the median variance of log R P , see Fig. 2c . This measure is equivalent to the median variance of log n S where n S is the number of stacking faults in the pillar provided that the stacking fault resistance R S is a constant, that is, R P = R S × n S (which is not perfectly true as we will show later). The median variance of log n S can be readily computed from the Poisson statistics, resulting from a random distribution with a mean value of n S = h / d S , where d S denotes the average stacking fault spacing, see solid lines in Fig. 2c . From the statistical analysis, one concludes that the average spacing between stacking fault defects is in the order of 4±1 nm, from which one derives a specific stacking fault resistance of . 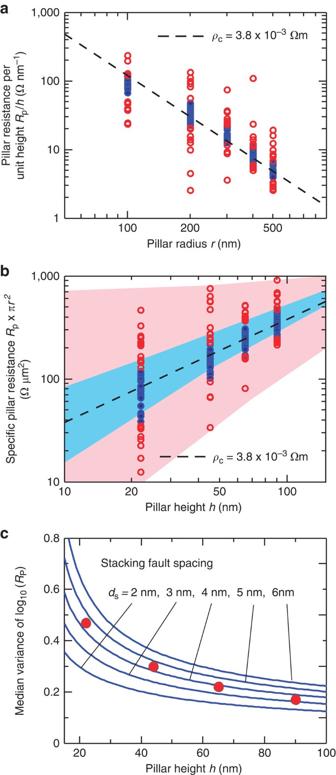Figure 2: Pillar resistance and data scatter analysis at low electric field strength. (a) Pillar resistance per unit heightRP/hversus pillar radiusrand (b) specific pillar resistanceRP× πr2versus pillar heighth. Data points are indicated by circular symbols and the full circles mark the data within the median variance band. Dashed lines: inverse quadratic (a) and linear (b) scaling according to equation (1) using the median value ofρc=3.8 × 10−3Ω m for the c-axis resistivity. The blue and red shaded bands inbshow the median variance band and the overall scatter of simulated data points for a mean stacking fault spacing ofdS=3.9 nm−1and specific stacking fault resistance ofrS=107±0.35Ω nm2. (c) Median variance of, full circles, versus pillar height determined from the data shown inb. Solid lines: same quantity computed from Poisson statistics for different values of the stacking fault spacingdSas indicated in the figure. Figure 2: Pillar resistance and data scatter analysis at low electric field strength. ( a ) Pillar resistance per unit height R P / h versus pillar radius r and ( b ) specific pillar resistance R P × π r 2 versus pillar height h . Data points are indicated by circular symbols and the full circles mark the data within the median variance band. Dashed lines: inverse quadratic ( a ) and linear ( b ) scaling according to equation (1) using the median value of ρ c =3.8 × 10 −3 Ω m for the c-axis resistivity. The blue and red shaded bands in b show the median variance band and the overall scatter of simulated data points for a mean stacking fault spacing of d S =3.9 nm −1 and specific stacking fault resistance of r S =10 7±0.35 Ω nm 2 . ( c ) Median variance of , full circles, versus pillar height determined from the data shown in b . Solid lines: same quantity computed from Poisson statistics for different values of the stacking fault spacing d S as indicated in the figure. Full size image The stacking fault spacing can be independently determined from the non-linearity of the I/V characteristics. A set of I/V curves measured for the 44-nm tall pillars is shown in Fig. 3a . An excellent fit to the data is obtained based on a one-dimensional thermally activated barrier model [16] , see dotted curves in Fig. 3a . We assume that a stacking fault defect can be represented electrically as a parabolic barrier Φ. The barrier acts as an energy filter for thermally excited charge carriers q . The transition probabilities in the direction of the electric field and in the reverse direction are exp(−(Φ− q Δ V /2)/ k B T ) and exp(−(Φ+ q Δ V /2)/ k B T ), respectively, where is the thermal energy at room temperature, and is the potential difference across the barrier. The total current across the barrier is proportional to the difference between the two transition rates. 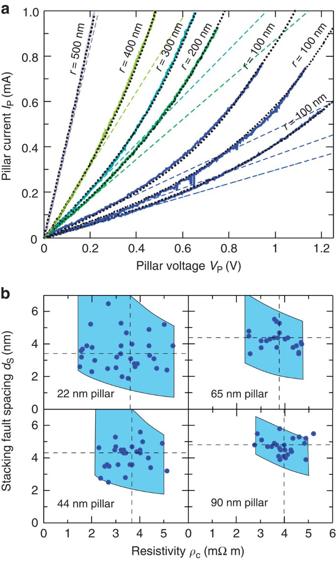Figure 3: Transport characteristics at high electric field. (a) Pillar current versus pillar voltage (I/V curves) for 44-nm tall pillars with radii of 100–500 nm as indicated in the figure: Dashed lines indicate the Ohmic conductance, 1/RP, at low bias, dotted lines correspond to a fit to the data using equation (2). Pillar resistanceRPand stacking fault spacingdSas determined from the fit are (from bottom-right to top-left curves): 3.53 kΩ/3.5 nm; 2.78 kΩ/4.7 nm; 2.11 kΩ/4.7 nm; 1.16 kΩ/4.5 nm; 0.96 kΩ/5.4 nm; 0.63 kΩ/6.2 nm and 0.23 kΩ/5.0 nm. (b) Stacking fault spacingdSversus c-axis resistivityρcobserved in pillars with a height of 22, 44, 65 and 90 nm. Data is only shown for whichρcis in the median variance band. Horizontal and vertical dashed lines correspond to the median valuesdSandρcin each panel, respectively. Shaded boxes show the area occupied by the respective parameters obtained from fitting simulated I/V curves. With Δ V = V P d S / h one finds (note that the model is mathematically equivalent to a one-dimensional barrier hopping model for localized trap states in a weak electric field [16] ) Figure 3: Transport characteristics at high electric field. ( a ) Pillar current versus pillar voltage (I/V curves) for 44-nm tall pillars with radii of 100–500 nm as indicated in the figure: Dashed lines indicate the Ohmic conductance, 1/ R P , at low bias, dotted lines correspond to a fit to the data using equation (2). Pillar resistance R P and stacking fault spacing d S as determined from the fit are (from bottom-right to top-left curves): 3.53 kΩ/3.5 nm; 2.78 kΩ/4.7 nm; 2.11 kΩ/4.7 nm; 1.16 kΩ/4.5 nm; 0.96 kΩ/5.4 nm; 0.63 kΩ/6.2 nm and 0.23 kΩ/5.0 nm. ( b ) Stacking fault spacing d S versus c-axis resistivity ρ c observed in pillars with a height of 22, 44, 65 and 90 nm. Data is only shown for which ρ c is in the median variance band. Horizontal and vertical dashed lines correspond to the median values d S and ρ c in each panel, respectively. Shaded boxes show the area occupied by the respective parameters obtained from fitting simulated I/V curves. Full size image where the exponential factor exp(−Φ/ k B T ) is implicitly contained in R P , and V P denotes the overall voltage drop across the pillar. The value of the stacking fault spacing d S , that is, the barrier spacing, is obtained by fitting the measured I/V data to equation (2). Figure 3b shows a scatter plot of the d S data from the fit versus corresponding resistivity ρ c values for the four pillar heights investigated. For better visibility, only data is shown for which ρ c is within the median variance band. The spread of d S correlates with the spread of ρ c and larger values of d S tend to correlate with smaller values of ρ c . We also note that the medians of d S and ρ c are systematically smaller in the short pillars than in the taller ones. The effect is most likely due to a systematic error, which is made in the evaluation of the spreading resistance R SP (see Methods section). Overall, the I/V curve fit yields a median value of the stacking fault spacing of , which is fully consistent with the corresponding value from the statistical analysis but significantly more precise. Simulation We performed a model simulation to better understand the origin of the statistical scatter in the data. At each stacking fault, the voltage drops abruptly by an amount, which according to equation (2) is given by where i P denotes the current density in the pillar. The stacking faults are randomly distributed over the graphite planes in the pillar with a uniform probability of , where 0.34 nm is the graphite layer spacing. In a second step the overall voltage drop is calculated using equation (3). In addition, we allow for random fluctuations of the barrier height. Correspondingly, we write r S = r S0 exp( U / k B T ), where U is a Gaussian random variable with zero mean and a s.d. ΔΦ. The parameter ΔΦ turns out to be important to correctly account for the scatter of the pillar resistance in Fig. 2b . For ΔΦ=0, the resistance fluctuation would be solely due to the Poissonian statistics of the stacking fault distribution in the pillar, which cannot account for the data points exhibiting a resistance which is substantially higher than the respective median values. However, excellent agreement with the measured data is obtained for ΔΦ=20 meV corresponding to a random variation of r S by a factor of 10 ±0.35 . The shaded bands in Fig. 2b show the spread of the specific pillar resistance obtained from 10,000 simulation runs, in which the specific defect resistance was adjusted to r S0 =10 7 Ω nm 2 to correctly reproduce the experimentally measured median resistivity of ρ c . The blue and red shaded bands indicate the median variance band and the overall spread of the simulated data, respectively. The bands from the simulation do not perfectly overlap with the corresponding data points from the experiment. This deviation is consistent with the statistical fluctuations expected from the size of the experimental data set, as was verified by analyzing simulation samples of comparable size. The simulation also correctly reproduces the correlation between the stacking fault spacing and the measured resistivity shown in Fig. 3b , in which the blue shaded boxes mark the area occupied by the parameters obtained from fitting the simulated I/V curves using exactly the same analysis procedure as the experimental data. The statistical analysis makes no assumptions on the transport mechanism and is therefore free of any model bias. Hence, the excellent agreement between the stacking fault distance determined from the statistical and the I/V data analysis provides significant evidence that at room temperature the physics of electrical transport along the c-axis is correctly captured by a thermally assisted barrier transport process. This is an intriguing unexpected finding in account of well-established theoretical concepts and experimental data, which, for example, reveal no evidence for a metal-insulator transition at low temperature. On the other hand, it has been proposed that an additional thermally activated channel could be responsible for the anomalous temperature dependence of ρ c , that is, an increase of the resistivity with decreasing temperature which is observed for temperatures >50 K (refs 4 , 7 ). From the published data in ref. 7 , one infers that the thermally activated transport dominates at room temperature, which is consistent with our experimental observations. The nature of the barrier is not clear at this point. It has been proposed that thermally activated barrier transport could proceed via localized Tamm states [4] . This view is supported by recent electronic structure calculations, which find two interface bands at stacking fault defects at an energy of above and below the Fermi energy [17] . The bands are not strict surface states but large amplitude resonances, which could act as efficient transfer channels across the stacking fault defect for thermally excited charge carriers. We can obtain a rough estimate of the barrier height from the measured specific stacking fault resistance r S0 . Given the mesoscopic pillar dimensions, we may assume coherence of the electron wave functions at the stacking fault interface, which allows us to use the Landauer–Buettiker formula [18] for estimating the overall transmission probability of the barrier , where n =38.2 nm −2 is the areal density of the atoms in a graphite plane. With h /2 q 2 =12.6 kΩ and r S0 =10 7 Ω nm 2 from the simulation, one obtains . Assuming that conduction states with an energy below the barrier height are essentially reflected at the stacking fault, that is, for E − E F <Φ, and states with an energy larger than the barrier height are perfectly transmitted, that is, for E − E F ≥Φ, one finds broadly consistent with the expected energy off-set of localized stacking fault states. The measured large value for the specific stacking fault resistance of r S =10 7±0.35 Ω nm 2 is orders of magnitude larger than the inter-layer resistance expected from a Drude model. This clearly demonstrates that close proximity of graphene sheets is not a sufficient condition for efficient current transport across the sheets, which in addition requires proper ABAB stacking. More importantly, we show that the stacking fault density, which in our case was in the order of 1 defect every 12th graphite sheet, can be determined from a simple transport experiment at least for samples with mesoscopic dimensions. This is a remarkable achievement since the stacking faults are very difficult to observe by standard x-ray and electron diffraction techniques due to the low scattering cross-section of carbon atoms and complications associated with the fabrication of suitable planar samples orthogonal to ab-axis. The fact that the dominant defect structure can be experimentally assessed in situ is a particularly valuable asset for the study of graphite-related transport phenomena in a wide context. Sample preparation High-quality HOPG ( μ mash, ZYA grade, 0.4 o mosaic spread) samples of centimetre size and with a thickness of ~2 mm were used as substrates. The cylindrical graphite pillars were fabricated from a freshly cleaved HOPG substrate by means of anisotropic oxygen plasma etching. In the first step, circular Pd/Au metal mesas were deposited onto the HOPG surface. On one hand, the metal mesas serve as electrical contacts of the top pillar surface and on the other hand as self-aligned etch-masks. They were fabricated by means of electron beam lithography and lift-off using a 100-nm thick PMMA resist layer. The metal mesas consist of 15 nm of Pd as adhesion promotor to the HOPG surface and 20 nm of Au as top layer and the metal layers were deposited by means of thermal evaporation. Prior to evaporation, a short oxygen plasma cleaning was applied to remove organic residues on the exposed HOPG surface. The pillar structures emerge during the plasma etch, which selectively thins down only the unprotected HOPG area. Reactive ion etching was performed on a Oxford Plasma Lab 80 plus tool. Oxygen pressure, 20 mbar, and bias potential, 200 V, were optimized to obtain a low etch rate of 11 nm min −1 for good control of the pillar height and to minimize chemical anisotropic side wall etching. Electron microscopy inspection of the fabricated pillars showed negligible under etching of the graphite pillars at the metal masks and only a minor side wall taper towards the HOPG substrate (see Fig. 1b ). Metal contacts of 8 × 8 arrays with radii of 100, 200, 300, 400 and 500 nm were written in 20 × 20-μm sized fields separated by 10 μm from each other. Pillars with a height of 22, 45, 65 and 90 nm were fabricated in a succession of four etch steps. The transport characteristics of a random selection of at least 10 pillars for every radius taken from at least two different fields were measured after each etch step. Measurements Measurements of the electrical transport on the structured HOPG sample were performed using a commercial AFM (Bruker Dimension V) at ambient conditions and using Pt/Ir-coated cantilever tips (Bruker SCM-PIT) with a spring constant of . The AFM also allows for the imaging and selection of the pillars for transport measurements. Electrical contact to the top surface of the pillars was established by cold welding the tip apex to the Au surface close to a centre position of the metal mesa by applying a vertical load force of and a current pulse of 1 mA for 1 s. The reproducible formation of the tip-metal contact was checked on a test sample consisting of an identical Pd/Au stack on an insulating glass substrate. The measured resistance which comprises the electrical resistance of the cantilever as well as the resistance of the actual tip apex to Au contact was R CL =270 Ω with a s.d. of ±9 Ω. This compound cantilever-contact resistance must be accounted for in the experiment as a corresponding series resistance. The electrical transport was characterized by measuring I/V characteristics. For this purpose, a potential V B of up to 2 V was applied to the cantilever tip using the voltage source of the AFM. The current flowing through the pillar, I P , was measured by means of a commercial virtual ground-type current-to-voltage converter (FEMTO DHPCA-100), which was connected to the sample stage via a series resistor R IL =1 kΩ to limit the maximum current to and via a passive 2nd order low pass filter with a cut-off frequency of 100 kHz to avoid overloading of the I/V converter by high frequency noise signals. The genuine voltage drop across the HOPG pillar is given by V P = V B − I P ( R IL + R CL + R SP ). The series resistance R SP =5.7 × 10 −5 Ω m/4 r where r denotes the pillar radius is due to the spreading resistance of the pillar to the HOPG substrate and it is inferred from the measured spreading resistance of Pd/Au contacts (see Spreading resistance section). I/V characteristics were measured up to a maximum current of I P =1 mA or a maximum voltage of V P =2 V × R P /( R P + R IL + R CL + R SP ), which ever occurred first. The pillar resistance R P = V P / I P is defined as the ratio of the pillar voltage divided by the pillar current. Spreading resistance The spreading resistance of the Pd/Au contacts on the HOPG substrate was measured prior to ion etching. The measured data were as expected for a classical diffusive transport model characterized by a 1/ r scaling, that is, , where the effective resistivity accounts for the large anisotropic electrical conductivity of the HOPG sample [19] , [20] . The values of the spreading resistance measured on different Pd/Au contacts of the same radius exhibit a substantial scatter of +100%/−50% with respect to the mean value. From a fit to a large data sample comprising at least 10 independent measurements for each contact radius, we obtained an effective resistivity of ρ eff =5.7 × 10 −5 Ω m ref. 21 . As shown in the paper, the c-axis resistivity inferred from the pillar resistance measurements is ρ c =3.8 × 10 −3 Ω m. Accordingly, one calculates an in-plane resistivity of ρ ab =8.55 × 10 −7 Ω m and a resistivity ratio of in agreement with the corresponding values cited in the literature for room temperature measurements. This confirms that the Pd/Au electrodes form an excellent low resistance contact to the HOPG surface. Important for our experiment is the penetration depth of the electric field into the HOPG sample along the c-axis. The penetration depth is given by , yielding 1.5 nm and 7.5 nm for the 100-nm and 500-nm radius pillars, respectively. To decouple genuine pillar transport properties from substrate effects, the pillar height must be larger than the penetration depth. Hence, the huge conductance anisotropy is a decisive factor, which enables the study of current transport on a length-scale that can reveal the stacking fault statistics. Data analysis A median analysis is used to cope with the expected non-Gaussian statistical scatter in the measurements. The standard mean value and variance are replaced by median and median variance measures, respectively, which are robust in the sense that they can be unequivocally measured independent from the underlying statistical model. The median separates the higher half of the data sample from the lower, and it corresponds to the value of a random variable at the 50% mid point of the cumulative distribution function. The median variance is defined here as the range spanned by 68% of the data, which are closest to the median corresponding to the range of a random variable with a cumulative probability in the interval from 16 to 84% in analogy to a Gaussian variance. I/V curve fit The measured I/V characteristics were fit to equation (1) retaining the pillar resistance R P and the stacking fault distance d S as free fit parameters and using the simplex search method implemented in the MATLAB function library. Error analysis The fabricated pillars can be readily imaged in the tapping mode, which allows the in situ measurement of the height and the radius of the HOPG pillars with a precision nm and nm, respectively. From equation (1), one finds that the error of the pillar resistance due to the pillar height uncertainty is corresponding to a relative error of and for a pillar height of h =22 nm and h =90 nm, respectively. Similarly, one finds for the error of the pillar resistance due to the radius uncertainty corresponding to a relative error of and for a pillar radius of r =100 nm and r =500 nm, respectively. In addition, the pillar cross-section is slightly tapered, see Fig. 1b , which is not accounted for in equation (1). Therefore, the pillar resistance is systematically overestimated inversely proportional to the pillar radius, which could explain the systematic deviation of the values from the scaling prediction observed in Fig. 2a for a pillar radius of 100 nm. In addition, we know from the simulation that similar deviations arise from statistical fluctuations due to the limited size of the data set. The most significant systematic error in the measurement of the pillar resistance is due to the spreading resistance R SP in the HOPG substrate. This is particularly an issue for the 22-nm tall pillars, which have a median resistance in the range from to for pillar radii of 100 nm and 500 nm, respectively. The spreading resistance itself exhibits a substantial relative variance of +100%/−50%. The magnitude of the variance is as expected given the uncertainty of the cantilever-contact resistance of ±9 Ω for contact radii >100 nm, whereas the origin of the variance for the smallest diameter contacts is unambiguously due to the HOPG substrate. The pillar resistance is computed from the measured total resistance V B / I P by subtracting the series resistances of R IL =1 kΩ for the current limiting resistor, R CL =270 Ω for the cantilever metal contact and R SP =5.7 × 10 −5 Ω m/4 r for the spreading resistance. By far, the biggest error arises from the spreading resistance term, in particular for low values of the pillar resistance. In all cases, the measured pillar resistance was larger than the calculated value for the spreading resistance, so we can be confident that the maximum error even for low resistance data points is always less than the deviation of the data point from the median value, which is the most important requirement for significance in the context of our work. How to cite this article: Koren, E. et al. Direct experimental observation of stacking fault scattering in highly oriented pyrolytic graphite meso-structures. Nat. Commun. 5:5837 doi: 10.1038/ncomms6837 (2014).